Hierarchical synthesis of non-centrosymmetric hybrid nanostructures and enabled plasmon-driven photocatalysis Non-centrosymmetric nanostructures consisting of multiple functional subunits represents an emerging class of hybrid nanostructures that can possess dramatic difference in property and functionality from concentric core–shell configuration. Here we develop a general synthetic method to achieve hierarchical control of high-order non-centrosymmetric hybrid nanostructures. The key is to employ a common intermedium for sequential conversion to all distinct predesigned subunits under similar growth condition, thus facilitating manifold control of a hybrid nanostructure. This advancement leads to an optimally designed plasmon-mediated photocatalytic nanostructure with 14.8-fold enhancement of photocatalytic efficiency as compared with conventional photocatalysts. Mechanistic study involving theoretical modelling and ultrafast time-resolved optical measurement uncovers a hot plasmonic electron-driven photocatalysis mechanism with an identified electron transfer pathway. This study may represent an important step towards high-level control of artificial nanostructures with new horizons for fundamental and technological applications. Hybrid nanostructures have become an important class of nanomaterials that can allow integration of distinct components (denoted as ‘subunits’) with different functionalities and have facilitated unique synergistic coupling effects [1] , [2] , [3] , [4] , [5] . As compared with concentric core–shell configuration whose surface chemistry is merely determined by the outermost shell component and is uniform [6] , [7] , non-centrosymmetric arrangement of functional subunits in a hybrid nanostructure (denoted as ‘ nc -HN’) can lead to new topological properties because each subunit can provide surface functional moieties with asymmetric synergistic coupling. This is of paramount significance for assembling and exploring new properties and can mimic oligomeric proteins in nature (for example, dimers, trimers and tetramers). For example, unique structural chirality can exist in a higher-order nc -HN because of its broken symmetry that is unattainable in its symmetric core–shell counterpart. Indeed, recent work has demonstrated the significance of controlling structural symmetry (from centrosymmetric to non-centrosymmetric configurations) of a simple two-component hybrid structure to its optical response as well as performance in water-splitting process [8] . However, controlled synthesis of the nc -HNs has not yet been fully explored that has led to limited applications. Most of available nc -HNs so far are limited to two-component heterodimers with conditioned-material combination. The major synthetic obstacle of high-quality complex nc -HNs originates from intrinsic chemical and structural incompatibility among different subunits, which has led to either poor material control (for example, limitation of material choice and polycrystallinity of semiconducting subunits) or unavailability of higher-order structures [3] . Thus, a more general synthetic approach that can allow the control of physical parameters in a predesignable nc -HN should be the key for creating novel and enhanced properties and may lead to applications in various fields. Herein we report a novel method to overcome long-term synthetic obstacles and to enable facile control of multifunctional higher-order nc -HNs. The complex nc -HNs that can incorporate catalytic, plasmonic, magnetic and semiconducting functionality with programmable composition, dimension and structural arrangement are reported, thus allowing investigation of their properties for versatile applications. This includes observation of plasmon-dependent enhancement of photocatalysis efficiency in a new family of nc -HNs. By combining theoretical modelling with elaborative material control, we elucidate the photocatalytic reaction pathway via a hot plasmon-induced electron transfer mechanism, which can be further confirmed by ultrafast time-resolved optical measurement. Unveiling the electron transfer pathway in a photocatalytic process may lead to a rational design of hybrid materials towards ultimate high quantum efficiencies as well as additional yet-unforeseen applications in other fields [9] , [10] , [11] , [12] , [13] , [14] . General synthetic scheme of high-order nc -HNs Most synthetic approaches of the nc -HNs so far are based on the epitaxial growth principle, typically requiring lattice matching as well as control of liquid–liquid or liquid–solid interfaces to sequentially expose facets of a nanoparticle to different chemical environments in order for epitaxial growth of targeted dissimilar subunits. In such growth processes, the interplanar lattice spacings of two neighbouring subunits are typically required to match at their intimate interface in order to avoid lattice strain and reduce energy for epitaxial nucleation and growth. One exemplary work is the growth of oxide semiconductor (Fe 3 O 4 )-based metal heterodimers (Fe 3 O 4 -Au and Fe 3 O 4 -Pt), in which a particular crystalline (111) plane is required at the interface of two subunits [15] , [16] . Similar heterodimers have also been achieved in metal–chalcogenides (for example, Au-CdSe, Au-CdS) with clear evidence of existence of epitaxial interface [17] , [18] . Recently, these resultant heterodimers have also been employed as seeds to further expose Au facets for stepwise epitaxial growth of other metal nanoparticles (for example, Ag, Ni, Pd and so on) to form higher-order nc -HNs [19] , [20] . However, all these epitaxy-based syntheses have limitation of material choice and cannot likely be scaled up for complex higher-order nc -HNs with multiple subunits and different structural arrangement [15] , [20] . Indeed, most studies of nc -HNs so far are mainly restricted to the simplest heterodimeric structures involving two subunits with constrained material choice, thus limiting their applications [15] , [16] , [17] , [18] , [19] , [20] , [21] , [22] , [23] , [24] , [25] , [26] , [27] . Under this context, a more general strategy that can allow to achieve complex high-order nc -HNs with adaptable combination and precise control of functional subunits is needed and should be the key for optimizing their property and related device performance. 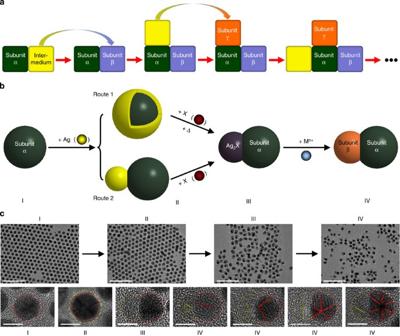Figure 1: Synthetic scheme for hierarchical and precise engineering of higher-ordernc-HNs. (a) Schematic key concept by utilizing a common intermedium for all targeted disparate subunits to develop a higher-ordernc-HN. (b) Two employed synthetic routes for integration and control of dual dissimilar subunits by using Ag as a common intermedium, in order to realize the synthetic concept ina. The chalcogenide compound M2n+Xnis used as an exemplary subunit β to depict the synthetic process but our approach can be readily extended to other types of subunits6. When the Ag is added to an existing subunit α (stage I), only two possible geometries can occur: core–shell (Route 1) and dimeric (Route 2) configurations (stage II). Both Route 1 and Route 2 can lead to a subunit α-amorphous Ag2X intermediate heterodimer (stage III). A targeted subunit β, M2n+Xn, can be achieved by ionic exchange of Ag2X with metal ions of Mn+(stage IV). (c,d) Demonstration of Route 1 synthesis for Au-CdSe heterodimers. Series of typical LR-TEM (c) and HR-TEM (d) images highlight different synthetic stages: (stage I) Au subunits; (stage II) AuAg core–shell; (stage III) Au-Ag2Se dimers; (stage IV) Au-CdSe heterodimers. Scale bar of LR-TEM images inc, 50 nm. Scale bar of HR-TEM images ind, 5 nm. In the HR-TEM images ind, dashed lines outline boundary of different components. Four different HR-TEM images of stage IV are presented, highlighting existence of various lattice orientations between Au and CdSe subunits without requirement of lattice match, which differs from an epitaxial structure (orange and red solid lines depict lattice orientation of CdSe and Au subunits, respectively). Figure 1a illustrates a novel synthetic concept with incorporation of a common intermedium for each targeted subunit in order to develop a predesigned higher-order nc -HN. A common intermedium is defined as a nanoparticle that can be utilized as a uniform template for adding all targeted subunits in a single nc -HN. As a result, instead of direct growth of a targeted subunit, a common intermedium is chosen and selectively added on existing subunits, followed by chemical transformations to a desired component. Figure 1: Synthetic scheme for hierarchical and precise engineering of higher-order nc -HNs. ( a ) Schematic key concept by utilizing a common intermedium for all targeted disparate subunits to develop a higher-order nc -HN. ( b ) Two employed synthetic routes for integration and control of dual dissimilar subunits by using Ag as a common intermedium, in order to realize the synthetic concept in a . The chalcogenide compound M 2 n+ X n is used as an exemplary subunit β to depict the synthetic process but our approach can be readily extended to other types of subunits [6] . When the Ag is added to an existing subunit α (stage I), only two possible geometries can occur: core–shell (Route 1) and dimeric (Route 2) configurations (stage II). Both Route 1 and Route 2 can lead to a subunit α-amorphous Ag 2 X intermediate heterodimer (stage III). A targeted subunit β, M 2 n + X n , can be achieved by ionic exchange of Ag 2 X with metal ions of M n + (stage IV). ( c , d ) Demonstration of Route 1 synthesis for Au-CdSe heterodimers. Series of typical LR-TEM ( c ) and HR-TEM ( d ) images highlight different synthetic stages: (stage I) Au subunits; (stage II) AuAg core–shell; (stage III) Au-Ag 2 Se dimers; (stage IV) Au-CdSe heterodimers. Scale bar of LR-TEM images in c , 50 nm. Scale bar of HR-TEM images in d , 5 nm. In the HR-TEM images in d , dashed lines outline boundary of different components. Four different HR-TEM images of stage IV are presented, highlighting existence of various lattice orientations between Au and CdSe subunits without requirement of lattice match, which differs from an epitaxial structure (orange and red solid lines depict lattice orientation of CdSe and Au subunits, respectively). Full size image In this new modular synthetic scheme, dimension and location of each subunit within an nc -HN are uniquely determined by its corresponding intermedium. Importantly, because the same intermedium can be applied for all distinct subunits residing in a higher-order nc -HN, sequential additions of dissimilar subunits can be achieved in an identical chemical environment, thus circumventing limitations imposed by distinct chemical and structural characteristics among ultimate subunits and making our approach feasible to scale up to more complex hierarchical hybrid nanostructures. An additional advantage of our new synthetic scheme includes that the judicious choice of chemical transformation based on Lewis acid–base reaction has been demonstrated to enable monocrystalline compound based on non-epitaxial growth mechanism [6] , which assures the exceptional quality of subunits without concern of interfacial lattice mismatching. Demonstration of addition of one subunit To detail our proposed synthetic scheme and highlight its unique control of subunits, Fig. 1b employs Ag as an example of common intermedium and illustrates step-by-step how a desired functional compound subunit can be adjoined on an existing one. While in general many other metals with soft Lewis acidity can be applied as an appropriate common intermedium, Ag is chosen in the current work based on two considerations. First, the growth of Ag nanostructures on a wide variety of seed nanoparticles has been extensively studied to generate either a conformal core–shell (Route 1) or a site-selective geometry (Route 2). The control of its dimension, location and morphology can be achieved by manipulating reaction kinetics [28] , [29] , [30] , [31] . Second, the high acid softness and electronegativity of Ag make it an appropriate element to facilitate various nanoscale chemical transformations, including the galvanic replacement of metals and cation exchange of compounds, which can offer a broad selection of targeted subunits [6] , [30] , [32] . Importantly, the synthetic process illustrated in Fig. 1b can be easily replicated stepwise to complete an nc -HN with a predesigned arrangement of its functional subunits by the sequential addition and control of the Ag intermedium. Figures 1c,d and 2 exemplify the key steps of the synthesis in Fig. 1b , quality of subunits and various controls of dimension and location that can be enabled by our approach, respectively. The generality and hierarchical control of more complex nc -HNs are presented in Fig. 3 by following the scheme in Fig. 1a . 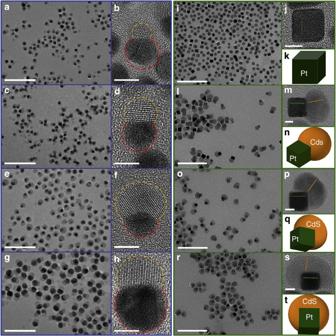Figure 2: Structural engineering of subunits. (a–h) Au-CdSe heterodimers with tunable sizes of both Au and CdSe subunits. (a,c,e,g) Typical LR-TEM images. Scale bar, 50 nm. Corresponding typical HR-TEM images are shown inb,d,f,h, respectively. Scale bar, 5 nm. Orange and red dashed curves outline dimensions of CdSe and Au subunits, respectively. (i–t) Pt-CdS heterodimers with controllable structural arrangement. (i,l,o,r) Typical LR-TEM images. Scale bar, 50 nm. Corresponding typical HR-TEM images are shown inj,m,p,s, respectively. Scale bar, 5 nm. Green and orange solid lines highlight lattice orientation of Pt and CdS subunits, respectively. Monocrystalline CdS subunits can be achieved in all structural configurations without requirement of lattice match between Pt and CdS that is enabled by non-epitaxial chemical transformation mechanism. (k,n,q,t) Structural model of Pt-CdS. Figure 2: Structural engineering of subunits. ( a – h ) Au-CdSe heterodimers with tunable sizes of both Au and CdSe subunits. ( a , c , e , g ) Typical LR-TEM images. Scale bar, 50 nm. Corresponding typical HR-TEM images are shown in b , d , f , h , respectively. Scale bar, 5 nm. Orange and red dashed curves outline dimensions of CdSe and Au subunits, respectively. ( i – t ) Pt-CdS heterodimers with controllable structural arrangement. ( i , l , o , r ) Typical LR-TEM images. Scale bar, 50 nm. Corresponding typical HR-TEM images are shown in j , m , p , s , respectively. Scale bar, 5 nm. Green and orange solid lines highlight lattice orientation of Pt and CdS subunits, respectively. Monocrystalline CdS subunits can be achieved in all structural configurations without requirement of lattice match between Pt and CdS that is enabled by non-epitaxial chemical transformation mechanism. ( k , n , q , t ) Structural model of Pt-CdS. 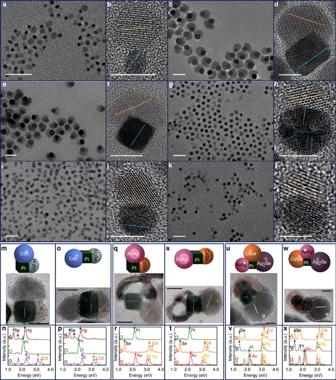Figure 3: Thenc-HNs with broad range of material combination and higher-order structural control. (a–l) LR-TEM and HR-TEM images of various heterodimers: FePt-CdSe (a,b), Pt-PbS (c,d), Pt-ZnS (e,f), Au-CdS (g,h), Au-PbSe (i,j) and Au-PbS (k,l). Scale bar of LR-TEM images, 50 nm; scale bar of HR-TEM images, 5 nm. Colour solid lines in HR-TEM images highlight lattice orientations of different subunits. (m–x) Higher-ordernc-HNs: Pt-CdS-HgSe (m–p), Pt-AuAg-CdSe (q–t) and Pt-Ag2Se-AuAg-CdSe (u–x). For each type ofnc-HN as shown, synthesis always starts with Pt nanocube as the first subunit, and every sequentially grown subunit is intentionally controlled to reside on only one facet of the Pt subunit in order to demonstrate structural control. As the Pt subunit has six identical surface facets, the third subunit can be grown either adjacent or opposite to the second subunit. As a result there are two different structures for each type ofnc-HN, as shown in the figures. This can further create important chirality of higher-ordernc-HNs of such as Pt-Ag2Se-AuAg-CdSe. For each type of higher-ordernc-HN, structural model and HR-TEM image (m,o,q,s,u,w) and single-point EDS recorded at the locations specified in corresponding HR-TEM images (n,p,r,t,v,x) are provided to support assignment of subunits. In HR-TEM images, colour-dashed curves outline boundaries of different subunits, and solid colour lines highlight lattice orientations of each subunit. Full size image Figure 3: The nc -HNs with broad range of material combination and higher-order structural control. ( a – l ) LR-TEM and HR-TEM images of various heterodimers: FePt-CdSe ( a , b ), Pt-PbS ( c , d ), Pt-ZnS ( e , f ), Au-CdS ( g , h ), Au-PbSe ( i , j ) and Au-PbS ( k , l ). Scale bar of LR-TEM images, 50 nm; scale bar of HR-TEM images, 5 nm. Colour solid lines in HR-TEM images highlight lattice orientations of different subunits. ( m – x ) Higher-order nc -HNs: Pt-CdS-HgSe ( m – p ), Pt-AuAg-CdSe ( q – t ) and Pt-Ag 2 Se-AuAg-CdSe ( u – x ). For each type of nc -HN as shown, synthesis always starts with Pt nanocube as the first subunit, and every sequentially grown subunit is intentionally controlled to reside on only one facet of the Pt subunit in order to demonstrate structural control. As the Pt subunit has six identical surface facets, the third subunit can be grown either adjacent or opposite to the second subunit. As a result there are two different structures for each type of nc -HN, as shown in the figures. This can further create important chirality of higher-order nc -HNs of such as Pt-Ag 2 Se-AuAg-CdSe. For each type of higher-order nc -HN, structural model and HR-TEM image ( m , o , q , s , u , w ) and single-point EDS recorded at the locations specified in corresponding HR-TEM images ( n , p , r , t , v , x ) are provided to support assignment of subunits. In HR-TEM images, colour-dashed curves outline boundaries of different subunits, and solid colour lines highlight lattice orientations of each subunit. Full size image Quality and size control of a subunit in nc -HNs Figure 1c shows one example of Au-CdSe heterodimers in great detail by following the Route 1 synthesis. By comparing with Au-CdSe heterodimers from the epitaxial growth method, one distinct feature of as-synthesized Au-CdSe heterodimers is that there is no lattice match between Au and CdSe subunits at their interface, while CdSe subunits sustain monocrystallinity that is independent of the lattice of Au subunits ( Fig. 1d ). This observation is supported by low-resolution (LR) and high-resolution (HR) transmission electron microscopy (TEM) and energy dispersive X-ray spectroscopy (EDS) characterization ( Supplementary Figs 1 and 2 ). It is worthy to note that the monocrystallinity of subunits is critical for the performance of final nc -HNs, particularly when defects become a limitation in the processes such as carrier recombination and transfer [33] , [34] . In the formation of Au-CdSe heterodimers, the intermedium Ag can be fully converted to the semiconductor CdSe without residue of Ag according to the EDS measurement ( Supplementary Fig. 1 ), and the size of the CdSe subunit is uniquely determined by that of the Ag intermedium, thus offering tunability and control of the dimension of subunits in an nc -HN. Figure 2a–h shows that sizes of Au and CdSe subunits can be independently tailored. As a result, our Au-CdSe heterodimers can be applied as a model system to explore finely tailored coupling between plasmons and excitons due to unique size-dependent excitonic and plasmonic characteristics ( Supplementary Fig. 3 ) [35] , [36] . Structural arrangement control of a subunit in an nc -HN In addition to fine control of its dimension, spatial arrangement of a subunit within an nc -HN should play a vital role in determining the synergistic coupling, which can also be achieved by our synthetic approach. We apply Pt-CdS heterodimers as an illustrative example because each Pt nanocube possesses six identical well-defined (100) facets ( Fig. 2i–k ) [37] . By simply manipulating growth kinetics of the Ag intermedium nanoparticles in a Route 2 synthesis, three distinct arrangements of CdS subunits can be achieved under otherwise similar synthetic condition: monocrystalline CdS subunits can reside on one, two and three adjacent facets of a Pt nanocubic subunit, respectively ( Fig. 2l–t and Supplementary Fig. 4 ). Material selectivity of subunits in nc -HNs Our method for control of monocrystallinity, dimension and structural arrangement of subunits in an nc -HN is very versatile and can be readily applied for a broad range of material selection, such as magnetic, catalytic, plasmonic and semiconducting subunits, to enable various synergistic couplings, with a few more heterodimeric examples demonstrated in Fig. 3a–l . Importantly, for all the nc -HNs, the monocrystalline feature of compound subunits is manifested without evidence of strain-induced lattice defects that is consistent with non-epitaxial growth mechanism, and further highlight the quality of subunit facilitated by our approach. Hierarchical control of subunits in an nc -HN Notably, all the controls demonstrated in Figs 1 and 2 offer the basis to form higher-order nc -HNs with structural and compositional tailoring by simply replicating the process. Figure 3m–x (see also Supplementary Figs 5 and 6 ) highlights examples involving three and four different functional subunits, respectively. As compared with symmetric core–shell nanostructures, higher-order nc -HNs are much more challenging to characterize because of their structural complexity and asymmetry. In particular, a typical TEM image only represents a two-dimensional (2D) projection of a nanostructure. Therefore, in addition to the LR-TEM imaging, we have employed angle-dependent TEM imaging, HR-TEM imaging and single-point EDS measurements to assign structure and evaluate uniformity and yield for each type of nc -HN (see Supplementary Figs 7 and 8 and Supplementary Note 1 ). Photocatalytic application of emerging nc -HNs It is worth noting that each subunit in a higher-order nc -HN can be independently tailored in a highly controllable manner similar to what has been demonstrated in Fig. 2 concerning important parameters such as composition, morphology and geometric arrangement. This offers tremendous opportunity to programme well-defined hybrid nanostructures with finely tuned synergistic coupling and to explore different fundamental chemistry and physics phenomena as well as novel technological applications at the nanoscale, which could be challenging otherwise. We choose a novel nc -HN family of Pt-Au x Ag 1− x -CdSe with tunable ratio x , in which both the plasmonic (Au x Ag 1− x ) and the monocrystalline semiconducting (CdSe) subunits occupy adjacent facets of a catalytically active subunit (Pt) with intimate interfacial contacts, respectively ( Fig. 4a ). The ratio x is defined as molar ratio of Au element in an AuAg alloy subunit. It is worthy to note that the structural model as well as HR-TEM images of Pt-Au x Ag 1− x -CdSe presented in Fig. 4 is intentionally chosen with a particular projection plane in order to clearly highlight individual subunits of an nc -HN. However, all subunits in this specific nc -HN family are confirmed to contact with each other by angle-dependent TEM imaging (see also Supplementary Fig. 7 and Supplementary Note 1 ), which therefore enhance synergistic coupling as well as facilitate transfer of charge carriers between subunits as discussed below. This type of nc -HN offers an example to examine finely tailored synergistic effects and to reveal new role of plasmons in photocatalysis that has not been settled in the field because of the lack of material control and predictive modelling [9] . 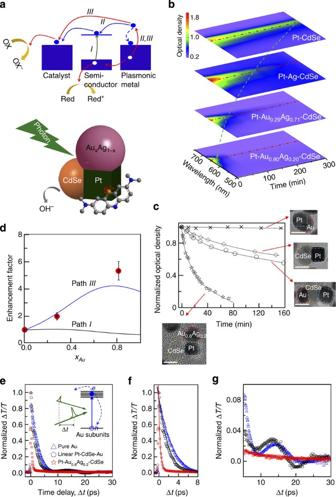Figure 4: Tailored plasmon-driven hot electron photocatalysis of the Pt-AuxAg1−x-CdSenc-HNs. (a) Schematicnc-HN and band diagram showing different conceivable reaction pathways of photocatalytic reduction of MB molecules by Pt-AuxAg1−x-CdSenc-HNs under visible light illumination. In our photocatalysis experiment, oxidizing (OX) and reducing (Red) agents are MB and ethanol molecules, respectively. (b) 2D time evolution of the optical absorption profile of the MB molecule enabled by Pt-AuxAg1−x-CdSenc-HNs with varying ratio ofx. An arrowed green dashed curve highlights the evolution of the photocatalytic reaction rate with the increase inxby comparing peak evolution at 677 nm (red dashed dot line). (c) Time-dependent normalized optical density of MB molecules at 677 nm with different well-designed photocatalysts. The optical density at different reaction time is normalized to the initial value before the photocatalytic reaction starts. (cross): Pt-Au; (diamond): Pt-CdSe; (pentagon): linear Pt-CdSe-Au; (star):Pt-Au0.80Ag0.20-CdSe. Corresponding typical HR-TEM images are provided for each curve. Scale bar, 10 nm. (d) Comparison of the theoretical and experimental dependence of enhancement factor of the photocatalytic reaction rate on the ratioxof annc-HN under excitation of 510 nm light. The error bars of experimental data points are derived by averaging enhancement factor from different batches of measurements and samples. (Blue curve): Theoretical enhancement via path III ina; (black curve): Theoretical enhancement via path I ina; (red solid circle): Experimental values. (e) Normalized optical transmission change (ΔT/T) as a function of time delay (Δt) in pump–probe measurements. The data show occurrence of intercorrelated energy transfer processes with different scattering interactions inside Au subunits. The inset ineshows schematic pump–probe process by exciting Au plasmon and detecting its electron decay at Δt. (f) Data excerpted frome, highlighting fast decay with single exponential fitting (solid curves). This regime can be attributed to energy exchange of electrons with lattice through electron–phonon coupling. (g) Data excerpted frome, highlighting possible impulsive excitation of coherent acoustic phonons. (Blue triangle): Pure Au nanoparticles; (black pentagon): linear Pt-CdSe-Au; (red star): Pt-Au0.8Ag0.2-CdSe. Figure 4: Tailored plasmon-driven hot electron photocatalysis of the Pt-Au x Ag 1− x -CdSe nc -HNs. ( a ) Schematic nc -HN and band diagram showing different conceivable reaction pathways of photocatalytic reduction of MB molecules by Pt-Au x Ag 1− x -CdSe nc -HNs under visible light illumination. In our photocatalysis experiment, oxidizing (OX) and reducing (Red) agents are MB and ethanol molecules, respectively. ( b ) 2D time evolution of the optical absorption profile of the MB molecule enabled by Pt-Au x Ag 1− x -CdSe nc -HNs with varying ratio of x . An arrowed green dashed curve highlights the evolution of the photocatalytic reaction rate with the increase in x by comparing peak evolution at 677 nm (red dashed dot line). ( c ) Time-dependent normalized optical density of MB molecules at 677 nm with different well-designed photocatalysts. The optical density at different reaction time is normalized to the initial value before the photocatalytic reaction starts. (cross): Pt-Au; (diamond): Pt-CdSe; (pentagon): linear Pt-CdSe-Au; (star):Pt-Au 0.80 Ag 0.20 -CdSe. Corresponding typical HR-TEM images are provided for each curve. Scale bar, 10 nm. ( d ) Comparison of the theoretical and experimental dependence of enhancement factor of the photocatalytic reaction rate on the ratio x of an nc -HN under excitation of 510 nm light. The error bars of experimental data points are derived by averaging enhancement factor from different batches of measurements and samples. (Blue curve): Theoretical enhancement via path III in a ; (black curve): Theoretical enhancement via path I in a ; (red solid circle): Experimental values. ( e ) Normalized optical transmission change (Δ T/T ) as a function of time delay (Δ t ) in pump–probe measurements. The data show occurrence of intercorrelated energy transfer processes with different scattering interactions inside Au subunits. The inset in e shows schematic pump–probe process by exciting Au plasmon and detecting its electron decay at Δ t . ( f ) Data excerpted from e , highlighting fast decay with single exponential fitting (solid curves). This regime can be attributed to energy exchange of electrons with lattice through electron–phonon coupling. ( g ) Data excerpted from e , highlighting possible impulsive excitation of coherent acoustic phonons. (Blue triangle): Pure Au nanoparticles; (black pentagon): linear Pt-CdSe-Au; (red star): Pt-Au 0.8 Ag 0.2 -CdSe. Full size image Nanoscale photocatalysis represents a promising route for harnessing an electromagnetic process to convert solar to chemical energies [11] , [38] , [39] , [40] . A typical nanoscale photocatalytic system exclusively involves semiconductor nanostructures, in which photogenerated electron–hole pairs in semiconductors can be rapidly separated at semiconductor–catalyst interfaces to perform redox chemistry at the catalytically active sites [3] , [9] , [11] , [41] , [42] . One current major challenge of semiconductor-based photocatalysis is the low-energy conversion efficiency because of small absorption coefficient, defect-induced fast carrier recombination and short carrier diffusion length, reflection loss by high refractive index, etc. While some of these issues can be remedied by improving sample quality (such as monocrystallinity of semiconductors as achieved in the current work), alternatively, a new concept of integrating plasmonic effects to enhance photocatalytic efficiency has been recently proposed with some compelling lines of evidence [10] , [43] . Nevertheless, the underlying enhancement mechanism, as well as the corresponding reaction pathway following optical excitation of plasmons, remains ambiguous. A predictive model combined with elaborative material control is necessary in order to gain an understanding of the upper limit of plasmon-mediated enhancement towards design of highly efficient photocatalysts [9] . To that, in order to evaluate and to compare the photocatalytic performance of new family of Pt-Au x Ag 1− x -CdSe nc -HNs with existing photocatalysts in literature [41] , [42] , we choose a standard redox reaction of methylene blue (MB) dye molecules as a model system, in which the MB molecules can be reduced to form colourless leucomethylene molecules upon addition of two electrons ( Fig. 4a and Supplementary Fig. 9 ). For conventional photocatalysts, such as Pt-CdSe heterodimers in former study [41] , a photo-induced electron–hole pair within CdSe nanoparticles can rapidly dissociate at the catalyst–semiconductor interface. The separated electrons then migrate through the catalytically active site of Pt towards the MB molecules for reduction (correspondingly, solvent molecules such as ethanol can act as organic hole scavengers to complete the redox reaction). As a result, the intensities of two characteristic absorption peaks of the MB molecules at 667 and 609 nm decrease with time, with a decay constant that is determined by the redox reaction rate ( Supplementary Fig. 10 and Supplementary Note 2 ). In order to validate our photocatalysis measurement and data analysis, we have first performed a control experiment by investigating the photocatalytic effect of as-synthesized Pt-CdSe heterodimers, and observed an efficiency comparable to former reports [41] , [42] , which provides the basis to further study enhancement in other higher-order nc -HNs ( Supplementary Table 1 and Supplementary Note 2 ). Importantly, we observe that when a plasmonic metal alloy subunit, Au x Ag 1− x , is coupled on the Pt-CdSe in a Pt-Au x Ag 1− x -CdSe nc -HN, the redox reaction rate can be significantly increased under the same light illumination condition ( Fig. 4b ). A clear dependence of the reaction rate on the ratio x of the Au x Ag 1− x subunits has been identified, and a maximally 14.8-fold enhancement was observed in the Pt-Au 0.80 Ag 0.20 -CdSe nc -HNs as compared with the photocatalytic reaction rate of the Pt-CdSe ( Supplementary Table 1 ). Structural characterization of nc -HNs before and after photocatalytic reactions suggests that all nc -HNs and their composition remain unchanged ( Supplementary Fig. 11 ). Mechanistic study of photocatalysis enhancement Significant enhancement of the photocatalytic reaction rate of Pt-Au x Ag 1− x -CdSe nc -HNs can be attributed to their unique structures and the resultant synergistic interaction among subunits according to a few key control experiments summarized as follows: first, all the nc -HNs that have demonstrated enhancement of photocatalysis efficiency are confirmed to have intimate contact among subunits. We have carefully characterized and determined both the structure and the composition of every nc -HN in this experiment by different techniques ( Supplementary Note 1 ). For example, using angle-dependent imaging, all subunits in the Pt-Au x Ag 1− x -CdSe nc -HNs are confirmed to contact with each other, which should facilitate synergistic coupling and the charge transfer process. Furthermore, elemental analysis confirms the composition of each subunit and eliminates the existence of impurities, such as chloride ions, that might complicate the photocatalytic process [44] . Second, we have observed that the reaction rate increases as the ratio of x increases at the constant illumination wavelength of 510 nm ( Fig. 4b ). This is consistent with the observation that localized surface plasmon resonance energy of alloyed Au x Ag 1− x nanoparticles can be monotonically tuned by its x ratio [45] . Third, for a specific nc -HN its wavelength dependence of the reaction rate shows agreement with its plasmonic resonance profile ( Supplementary Fig. 12 ). We have systematically carried out illumination wavelength-dependent measurements for an nc -HN with fixed ratio x , and the result suggests that our observed photocatalysis enhancement is indeed related to the optical excitation of localized plasmon resonance of Au x Ag 1− x subunits. Last, the absence of synergistic coupling shows no enhancement of the photocatalytic reaction rate. We have performed similar photocatalytic measurements with two different mixtures of 1:1:1 molar ratio of Au, Pt and CdSe nanoparticles and 1:1 molar ratio of Au-Pt heterodimers and CdSe nanoparticles; however, we have not observed any enhancement of photocatalytic reaction rate from both samples ( Fig.4c ; and Supplementary Fig. 13 ). In order to elucidate the role of plasmonic subunit in a photocatalytic process and the underlying enhancement mechanism of photocatalysis presented in the Fig. 4b,c , Fig. 4a illustrates different mechanisms with three possible electron transfer pathways in the Pt-Au x Ag 1− x -CdSe nc -HNs under visible light illumination. Path I shows direct electron–hole pair excitation and dissociation from the semiconductor subunits followed by electron and hole transfer to catalysts and organic hole scavengers in solution, respectively. In this mechanism, the photon absorption of semiconductor subunits is enhanced by the neighbouring plasmonic subunit (that is, near-field electromagnetic enhancement) [34] , [36] , [46] . Paths II and III originate from excitation in the plasmonic metal subunits. In addition to the near-field electromagnetic enhancement effect, the optically excited plasmons of metal nanoparticles can quickly (within a few picoseconds) dissociate into hot electron carriers in the Fermi sea before a phonon-induced thermal equilibrium is reached [33] , [47] . Such energetic carriers have been recently demonstrated to be able to cross high-energy potential barriers [13] , [48] , [49] . Given the geometric arrangement of subunits in the Pt-Au x Ag 1− x -CdSe nc -HNs, paths II and III represent two possible transfer sequences once the hot plasmonic electrons are created: one involves available conduction states of semiconductor subunits to bridge electron transfer from the metallic to catalytic subunits (path II) and the other follows a direct transfer from the metallic to catalytic subunits (path III). For both pathways, the semiconductor subunits are needed in order to mediate hole transfer to the organic solvent to complete a redox reaction. In order to evaluate the validity of the above three reaction pathways in our observation of photocatalysis enhancement, we have combined our achieved fine materials engineering of nc -HNs ( Fig. 4c , and Supplementary Figs 14 and 15 ) with the development of a plasmon–photocatalytic model by considering both electron transfer and near-field electromagnetic enhancement mechanisms ( Fig. 4d ; Supplementary Figs 16–19 and Supplementary Note 3 ). To compare with our modelling, we have determined the photocatalysis enhancement of different nc -HNs (possessing different x ratio) by normalizing their reaction rate to that of Pt-CdSe heterodimers, with a summary presented in the Fig. 4d (see also Supplementary Table 1 and Supplementary Note 2 ). In our model, one main assumption is that the generation of electron–hole pairs in the semiconducting and plasmonic subunits is the driving mechanism of the photocatalysis and the photogenerated electrons can be transferred to the catalytic subunits, which is supported by the fact that the photocatalytic activity appears when we incorporate the CdSe and Au x Ag 1− x subunits ( Supplementary Figs 10, 13 and 15 ) to the Pt subunits. Importantly, the removal of electrons from the system to accomplish the reduction should be accompanied by the removal of holes since the system should be neutral to remain active. This hole transfer process typically requires a relatively large population of photoexcited holes in the Au x Ag 1− x subunits, and indeed recent work has predicted a large number of energetic holes in the d -band, which can facilitate carrier transfer to the CdSe subunits (again, our experimental confirmation on the interfacial contact between the Au x Ag 1− x and CdSe subunits by angle-dependent imaging supports the possibility for such hole transfer process, as revealed in Supplementary Fig. 8 ) [50] , [51] . As a result, the reaction rate is proportional to the total absorption cross-section of these subunits , where and are the absorption cross-sections of the Au x Ag 1− x and CdSe subunits within a Pt-Au x Ag 1− x -CdSe nc -HN, respectively. This can allow us to evaluate the photocatalysis enhancement by and to compare with our experimental data, where and represent the reaction rate and absorption cross-section of CdSe subunit within a Pt-CdSe heterodimer, respectively. We first evaluate path I under consideration of non-radiative energy transfer from metal plasmons to semiconductor excitons because of the localized intense electromagnetic field in the proximity of a photoexcited plasmonic nanostructure [34] , [45] , [52] . While this mechanism can indeed lead to maximally ~1.25-fold enhancement when compared with that of Pt-CdSe heterodimers ( Supplementary Note 3 ), it does not agree with our two key experimental observations: first, the Pt-Au 0.8 Ag 0.2 -CdSe nc -HNs exhibit a 14.8-fold enhancement of photocatalytic efficiency compared with the Pt-CdSe, which is much larger than the predicted enhancement. Second, the enhancement factor shows dependence on the ratio of x ( Fig. 4d ), suggesting that this mechanism could not play the dominant role. To differentiate paths II and III as well as to highlight the importance of the hierarchical structure of nc -HNs for photocatalytic performance, we have performed one important control experiment by synthesizing a linear type of nc -HNs with Au and Pt subunits physically separated by the semiconducting CdSe subunit in the middle ( Fig. 4c and Supplementary Fig. 14 ). As the plasmonic and catalytic subunits no longer have intimate contact, only path II can be allowed in this linear nc -HN. We have performed photocatalysis measurements under same condition with linear nc -HNs. The result shows significantly smaller photocatalysis efficiency as compared with those of the nc -HNs with all three subunits intimately contacted ( Fig. 4c ). This control experiment can therefore safely rule out path II as the main contribution to our observed enhancement in the Fig. 4d , and path III should be the prevailing hot electron transfer sequence in the photocatalytic reaction. Qualitatively, the efficiency difference between paths II and III can be understood by the fact that path III does not require hot electrons to pass through an interfacial semiconductor barrier. However, the semiconducting subunit plays an indispensible role in the process as a hole scavenger, as evidenced by another control experiment involving photocatalytic measurement of Pt-Au heterodimers (that is, absence of CdSe subunit) under same condition. We have not yet observed an efficient photocatalytic response from the Pt-Au heterodimers ( Fig. 4c and Supplementary Fig. 13 ), which provides a strong argument for our mechanism (path III) based on the hole transfer process to the semiconducting subunits. Importantly, this new mechanism of plasmon-driven hot electron photocatalysis can be further supported by our model (blue curve in the Fig. 4d and see also Supplementary Note 3 ). From our model, we can see that the plasmonic subunits can indeed provide such enhancement with similar dependence on the x ratio and the calculated enhancement factor following path III indicates a maximum factor of . This calculation is in reasonable agreement with the experimental observation. To further experimentally confirm this hot electron transfer scenario, we have performed ultrafast time-resolved optical spectroscopy measurement under photocatalytic condition on three control samples with finely tailored structural configurations. As outlined in our proposed model in Fig. 4a , high photocatalysis efficiency requires the electrons to be transferred to the catalytically active metal (for example, Pt subunits here) while competing with charge recombination and defect trap states. In all our time-resolved experiments ( Supplementary Fig. 20 ), pump and probe energies are tuned to directly excite plasmons and detect the temporal evolution of hot electrons within the Au subunits of nc -HNs, respectively (inset of Fig. 4e ). The results are summarized in Fig. 4e–g . Three control samples manifest dramatic differences in hot electron dynamics within the Au subunits. For pure Au nanoparticles, the hot electrons decay with an ~5 ps timescale through electron–phonon coupling. Since there is no channel for electron transfer in pure Au nanoparticles, energy deposited in electrons by pump pulses can be subsequently transferred to phonon modes with observation of a clear periodic oscillation modulation that can be attributed to acoustic phonon vibration of Au ( Fig. 4g , see also Supplementary Note 4 ) [33] , [53] , [54] . When the Au subunit is coupled to other subunits in an nc -HN, relaxation process of charge carriers (as well as associated energy flow) in Au can be significantly modified because of possible electron transfer between subunits. In particular, for the Pt-Au 0.8 Ag 0.2 -CdSe nc -HNs with intimate contact between metallic and catalytic subunits, we have observed a significant reduction of the decay constant to 0.32 ps as compared with 2.61 ps in pure Au nanoparticles, indicating that most hot electrons are transferred to the Pt subunits ( Fig. 4f ). Further comparison with the decay constant in linear Pt-CdSe-Au (2.02 ps) suggests that hot electron transfer in the Pt-Au 0.8 Ag 0.2 -CdSe nc -HNs occurs mainly between Pt and Au subunits because of their low interfacial energy barrier. Another strong piece of evidence for efficient hot electron transfer between Au and Pt subunits in the Pt-Au 0.8 Ag 0.2 -CdSe nc -HNs is the complete absence of acoustic phonon excitation after plasmon excitation, which is different from observations in both pure Au nanoparticles and linear Pt-CdSe-Au structures ( Fig. 4g ). This can be understood that the pump pulses energy deposited to the plasmonic excitation of Au subunits can be efficiently transferred to the Pt subunits via hot electron transfer. As a result, there is no enough energy residing in the Au subunits to impulsively excite their phonon modes. While more in-depth ultrafast spectroscopy measurements in conjunction with rate equation calculation should be needed in order to quantize the hot electron transfer process (and is currently under investigation), our results in Fig. 4e–g clearly confirm hot electron transfer process depicted in Fig. 4a . From the materials’ viewpoint, as compared with all former plasmonic photocatalytic systems, including the Au-TiO 2 with controversial photocatalysis enhancement mechanisms [55] , [56] , our Pt-Au x Ag 1− x -CdSe nc -HNs possess tunable plasmonic and semiconducting subunits with well-defined intimate interfacial contact with catalytic subunits. Such nc -HNs provide explicit evidence of the requirement of hot energetic electrons in order to achieve strongly enhanced photocatalysis. The agreement between our model and controlled experiments has further supported the hot plasmonic electron-assisted photocatalysis mechanism through path III in Fig. 4a . Our study immediately opens up exciting unforeseen opportunities, ranging from multifunctional nature-mimicking nanoscale oligomeric structures to a wide range of enabled applications. Our versatile modular synthetic method not only leads to high-quality and precise engineering of nc -HNs (including compositions, dimensions and structural arrangements) but also allows hierarchical growth of complex nc -HNs with flexible material choice, thus enabling novel synergistic functionality in a predesigned structure for both fundamental understanding and technology applications. For example, by maneuvering structural arrangement of subunits in an nc -HN (as demonstrated in the current work), the interfacial energy barrier between subunits can be controlled and utilized to guide the charge carrier flow path, which should be critical for various device concepts [13] , [14] . Importantly, through the combination of a new type of plasmon-photocatalytic nc -HNs with theoretical modelling and an ultrafast optical study, energetic plasmon-driven electrons are demonstrated to direct a photocatalytic process, and thus play a key role in the catalytic enhancement. The elucidation of different roles of plasmonic metals, semiconductors and catalysts in a photochemical reaction puts the requirement on the nanoscale design, in which the plasmonic, semiconducting and catalytic subunits must have a common transparent interface. It can thus allow us to evaluate a possible upper limit of a plasmon-assisted photocatalytic reaction and guide the design towards highly efficient structures. While our current study utilizes reduction/oxidation of MB molecules as an example to demonstrate plasmon-assisted catalytic enhancement, related hot electron physics uncovered in our work should be a general process under photoexcitation, as long as materials and interfacial coupling among functional subunits are taken into account to minimize the energy barrier for facilitating hot electron transfer. This should allow us to explore other nc -HNs desirable for different photoreactions, including water splitting and sensors [9] , [10] , [11] , [12] , [13] , [14] . Synthesis of nc -HNs All nc -HNs are synthesized in solution phase with chemicals as received without further processing. All aqueous solutions and related photocatalytic measurements are prepared in deionized water with resistivity of 18.3 MΩ cm (using the Barnstead NANOPure water purification system). Details of the synthetic procedure for the individual nc -HNs can be found in the Supplementary Methods . Structural and morphological characterization Samples for TEM characterization are prepared by adding one drop of solution with product onto a 300-mesh copper grid with carbon support film (Ted Pella no. 01820). JEOL 2100F and JEM 2100 LaB6 TEMs are used for all images presented in this work. Single-point EDS measurements are operated under scanning transmission electron microscopy mode using the JEOL 2100F. As a typical higher-order nc -HN can possess complex structure and a TEM image represents only a 2D projection of structure, we have carefully performed single-point EDS and angle-dependent imaging of every species of nc -HNs presented in order to confirm their structural configuration. Photocatalysis measurements All photocatalytic experiments are performed in a homemade apparatus, equipped with a Nikon super-high pressure Mercury lamp (150 W) and external lens pairs for collimation and control of beam size. A set of interference filters (full-width at half-maximum ~10 nm) from Newport Corp and Thorlabs Inc are applied to determine illumination wavelength, and a variable metallic neutral density filter wheel is used to allow accurate adjustment of illumination intensity. The photocatalytic experimental procedure is adapted from published methods [41] , [42] . All absorption spectra presented in this work are recorded by a commercial spectrophotometer (UV-2501PC, Shimadzu). The reaction rate in a photocatalytic process is evaluated by fitting the time-dependent absorption profile with a single exponential function. The normalized enhancement factor in Fig. 4d is determined by normalizing the reaction rate of different samples to that of the Pt-Ag-CdSe nc -HNs (see also Supplementary Note 2 ). Ultrafast time-resolved optical spectroscopy All ultrafast time-resolved experiments are performed at room temperature under photocatalysis condition in a 1-mm-thick fused silica liquid cell (Starna Cells). Two independent homemade optical parametric amplifers with a 250-kHz repetition rate are applied for pump–probe measurements ( Supplementary Fig. 20 ). The pump and probe energies are tuned to 2.51 eV. A typical pump power is 1 mW, and the probe intensity is attenuated by ~15 times. In order to increase detection sensitivity for such an acoustic phonon vibration, a laser power stabilizer with feedback control is added into the probe beam to reduce static noise level. The output laser pulses are further compressed by prism pairs to produce pulse width less than 100 fs. The time evolution of Δ T/T measured by the probe directly reflects the absorption change induced by the laser pump pulse. Theoretical modelling For theoretical calculations, the DDA code is taken from open source code at http://www.astro.princeton.edu/~draine/DDSCAT.html . Further details of modelling are given in Supplementary Note 3 . How to cite this article: Weng, L. et al. Hierarchical synthesis of non-centrosymmetric hybrid nanostructures and enabled plasmon-driven photocatalysis. Nat. Commun. 5:4792 doi: 10.1038/ncomms5792 (2014).